Cytosine methylation regulates oviposition in the pathogenic blood flukeSchistosoma mansoni Similar to other metazoan pathogens, Schistosoma mansoni undergoes transcriptional and developmental regulation during its complex lifecycle and host interactions. DNA methylation as a mechanism to control these processes has, to date, been discounted in this parasite. Here we show the first evidence for cytosine methylation in the S. mansoni genome. Transcriptional coregulation of novel DNA methyltransferase (SmDnmt2) and methyl-CpG-binding domain proteins mirrors the detection of cytosine methylation abundance and implicates the presence of a functional DNA methylation machinery. Genome losses in cytosine methylation upon SmDnmt2 silencing and the identification of a hypermethylated, repetitive intron within a predicted forkhead gene confirm this assertion. Importantly, disruption of egg production and egg maturation by 5-azacytidine establishes an essential role for 5-methylcytosine in this parasite. These findings provide the first functional confirmation for this epigenetic modification in any worm species and link the cytosine methylation machinery to platyhelminth oviposition processes. Schistosomiasis is one of the most important neglected tropical diseases afflicting humans, when viewed in terms of its prevalence, negative impact on disability adjusted life years (a metric for measuring morbidity) [1] and annual mortality rates [2] . More than 200 million people suffer from this chronic and debilitating disease, with 90% of all worldwide cases arising in poverty-stricken areas of sub-Saharan Africa [3] . Praziquantel is the current drug of choice to treat schistosomiasis, but the need for repetitive treatment in endemic communities, concerns over the emergence of drug resistance and an unknown mechanism of action [4] have all catalysed an urgent search for new chemotherapeutic agents. Three major blood fluke species within the phylum Platyhelminthes, genus Schistosoma ( S. japonicum , S. haematobium and S. mansoni ), cause schistosomiasis in humans. Largely restricted to Africa, South America, the Middle East and the West Indies, S. mansoni infection is initiated when humans are exposed to fresh water harbouring free-swimming cercariae. On percutaneous invasion of the definitive human host, schistosomes undergo complex developmental reprogramming necessary for survival in a hostile new environment, as well as to facilitate migration to the vasculature surrounding the bowels. Notable characteristics of this process include the complete transformation of surface membranes [5] , the dependence on haematophagy as a major energy source, the selective de novo expression of several hundred gene products [6] and the differentiation into morphologically and transcriptionally distinct adult male and female pairs [7] capable of producing hundreds of eggs every day. The host's immune response and microspines covering the eggshell surface facilitate the transendothelial passage of eggs into the intestinal lumen from where they are released with faeces. On contact with fresh water, the eggs hatch into ciliated miracidia capable of locating and infecting a suitable intermediate snail host (genus Biomphalaria ). Within the snail, miracidia shed their ciliated plates and develop into asexually reproducing sporocysts that ultimately release human-infective cercariae. Unfortunately, many of the eggs produced in the human host remain trapped in the intestinal wall or are swept back into the liver where they provoke a vigorous immune-mediated, circumoval granulomatous response resulting in peri-portal and hepatic fibrosis. It is the collective effect of these egg-induced reactions that, almost exclusively, lead to the development of pathology, morbidity and mortality associated with infection. Understanding the molecular mechanisms underpinning schistosome developmental maturation into egg-laying adult worm pairs are consequently of paramount importance in our search for novel anthelmintic targets, drugs and strategies. In the only previous study surveying for DNA methylation in S. mansoni , Fantappie et al . [8] did not detect any evidence for either adenine or cytosine methylation. This finding was surprising as the schistosome genome contains several characteristics [9] associated with methylation (for example, under representation of CpG sites and composition of 40% repetitive elements). Nevertheless, the observations of Fantappie et al . were concordant with several previous investigations that all failed to identify a functional role for DNA methylation in any worm species [10] . Prima facie , these reports imply that DNA methylation does not appear in the schistosome genome or feature as a control mechanism during parasite development and host interactions. However, there is now growing evidence for the presence of DNA methylation in many invertebrates, with 5-methylcytosine (m5C) detected in cnidarians (for example, Hydra [11] ), molluscs (for example, Donax trunculus [11] ), urochordates (for example, Ciona intestinalis [12] ), arthropods (for example, Drosophila melanogaster [13] ), echinoderms (for example, Echinus esculentus [14] ) and annelids (for example, Chaetopterus variopedatus [15] ). Unlike the developmental roles ascribed for DNA methylation in vertebrates (X chromosome inactivation [16] , allelic exclusion [17] , gene regulation [18] , embryogenesis [19] and repetitive element silencing [20] ), the function of this epigenetic regulator at the vertebrate/invertebrate boundary is less clearly defined. As schistosomes represent a derived invertebrate lineage, any information related to the identification and function of DNA methylation within these acoelomate organisms may well shed light on its contributory role during early bilateria evolution. Here we demonstrate that the S. mansoni genome is epigenetically modified and that parasite developmental maturation is linked to quantifiable changes in DNA methylation. Although previous studies have failed to identify a functional role for cytosine methylation in any examined worm species [10] , we provide evidence that this epigenetic modification is found associated with repetitive genomic elements and also regulates the important process of schistosome oviposition and egg development. It is anticipated that our results may provide new targets for schistosomiasis control, as well as fascinating insights into the early events of metazoan evolution by suggesting a critical role for cytosine methylation in the development of bilateral symmetry, sexual reproduction and organogenesis. The S. mansoni genome is methylated We used a selection of biophysical, molecular, immunological and cytochemical methodologies to survey for the presence of m5C (the most common methylated metazoan nucleobase [21] ). This comprehensive approach was chosen to minimize false conclusions about the methylation status of the schistosome genome, to apply more sensitive techniques than used by Fantappie et al . [8] and to maximize the certainty of detection. Examination of RNA-free, mixed-sex adult schistosome genomic DNA (gDNA) using gas chromatography coupled to mass spectrometry (GC–MS) yielded the first evidence of m5C ( m / z =296.2, retention time=15.70 min) in this species ( Fig. 1a ). We subsequently extended this observation to other schistosome lifecycle stages (including eggs, miracidia, sporocysts, cercariae, schistosomula and sexually mature male and female worms) by employing immunological detection of m5C using enzyme-linked immunosorbent assay (ELISA; Fig. 1b ). Here, all assayed schistosome developmental forms (free from host contamination, for example, Mus musculus gDNA) contained detectable, but variable, levels of m5C within their genome complements. To further demonstrate that the detected schistosome m5C was present within nuclear compartments, immuno-cytochemical assays (immunolocalization/genome in situ hybridisation (GISH)) were performed on cytological spreads obtained from schistosome infected Biomphalaria glabrata snails. Here, m5C was detected in nuclei derived from both the intra-molluscan sporocyst cells (Sm—blue, red and green nuclei, Fig. 1c ) and B. glabrata cells (Bg—blue and green nuclei, Fig. 1c ). These data (m5C positively stained sporocyst nuclei) clearly confirmed the ELISA results ( Fig. 1b ). Moreover, in addition to the central S. mansoni observation, immuno-cytochemical detection of m5C provided the first evidence for this form of epigenetic modification in the intermediate molluscan host, B. glabrata . 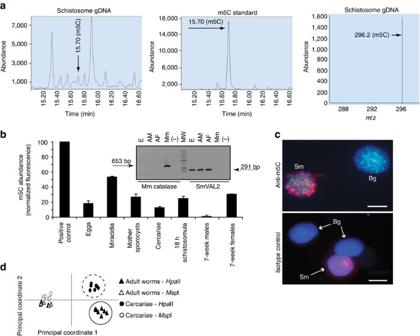Figure 1:Schistosoma mansonicontains a methylated genome. (a) GC–MS identification of m5C from mixed-sex, adult schistosome gDNA (compared with m5C standard). Selective ion-monitoring (m/z=296.2) by MS confirmed the presence of m5C in schistosome gDNA (right panel), which corresponded to an eluted GC peak at 15.7 min (left and middle panel). (b) ELISA detection of m5C across the schistosome lifecycle. Histograms (+, s.d.) represent mean m5C abundance (n=2 for each lifecycle stage), which was normalized (to both positive and negative control DNA samples). Data are representative of two independent experiments. Inset: agarose gel illustrates that schistosome gDNA isolated from life stages resident in the definitive host (E, egg; AM, adult male; AF, adult female) were not contaminated byM. musculus(Mm) gDNA. Primers designed to amplifyM. musculus(Mm) catalase (653 bp product, solid arrow, NCBI accession number X52108.1) andS. mansoni(Sm) Venom Allergen Like (VAL) 2 (291 bp product, dashed arrow, NCBI accession number AY994062.1) were used. (−) represents PCR conditions when no gDNA was included and MW represents molecular weight standards. (c) m5C immunolocalization/GISH analysis of cytological spreads derived fromS. mansoni(Sm) infectedB. glabrata(Bg) snails. Anti-mouse m5C (IgG1) and isotype control (murine IgG1) primary antibodies were detected by Alexa Fluor 488 F(ab')2goat anti-mouse IgG (H+L) secondary antibodies (green) during immunolocalization, whereas rhodamine (red)-labelled Sm gDNA was used to detect Sm nuclei during GISH. 4,6-Diamidio-2-phenylindole (blue) was used as a counter stain to identify both Bg and Sm nuclei. Scale bar, 2 μm. (d) MSAP analysis of m5C in gDNA obtained from cercariae and adult worms.HpaII (filled shapes) andMspI (open shapes) isoschizomers were used to restrict mixed-sex adult worm (triangles) and cercariae (circles) gDNA samples. Seven replicate samples were analysed for both schistosome life stages. MSAP data is illustrated by principal coordinate analysis.HpaII loci enclosed by a dashed circle represent m5C identified in cercariae andHpaII loci enclosed by a solid circle represent m5C identified in adults. Figure 1: Schistosoma mansoni contains a methylated genome. ( a ) GC–MS identification of m5C from mixed-sex, adult schistosome gDNA (compared with m5C standard). Selective ion-monitoring ( m / z =296.2) by MS confirmed the presence of m5C in schistosome gDNA (right panel), which corresponded to an eluted GC peak at 15.7 min (left and middle panel). ( b ) ELISA detection of m5C across the schistosome lifecycle. Histograms (+, s.d.) represent mean m5C abundance ( n =2 for each lifecycle stage), which was normalized (to both positive and negative control DNA samples). Data are representative of two independent experiments. Inset: agarose gel illustrates that schistosome gDNA isolated from life stages resident in the definitive host (E, egg; AM, adult male; AF, adult female) were not contaminated by M. musculus (Mm) gDNA. Primers designed to amplify M. musculus (Mm) catalase (653 bp product, solid arrow, NCBI accession number X52108.1) and S. mansoni (Sm) Venom Allergen Like (VAL) 2 (291 bp product, dashed arrow, NCBI accession number AY994062.1) were used. (−) represents PCR conditions when no gDNA was included and MW represents molecular weight standards. ( c ) m5C immunolocalization/GISH analysis of cytological spreads derived from S. mansoni (Sm) infected B. glabrata (Bg) snails. Anti-mouse m5C (IgG 1 ) and isotype control (murine IgG 1 ) primary antibodies were detected by Alexa Fluor 488 F(ab') 2 goat anti-mouse IgG (H+L) secondary antibodies (green) during immunolocalization, whereas rhodamine (red)-labelled Sm gDNA was used to detect Sm nuclei during GISH. 4,6-Diamidio-2-phenylindole (blue) was used as a counter stain to identify both Bg and Sm nuclei. Scale bar, 2 μm. ( d ) MSAP analysis of m5C in gDNA obtained from cercariae and adult worms. Hpa II (filled shapes) and Msp I (open shapes) isoschizomers were used to restrict mixed-sex adult worm (triangles) and cercariae (circles) gDNA samples. Seven replicate samples were analysed for both schistosome life stages. MSAP data is illustrated by principal coordinate analysis. Hpa II loci enclosed by a dashed circle represent m5C identified in cercariae and Hpa II loci enclosed by a solid circle represent m5C identified in adults. Full size image We next sought to evaluate whether changes in cytosine methylation associated with developmental progression could be influenced by different environmental challenges. For this, we used a genome-wide approach, methylation-sensitive amplification polymorphism (MSAP) [22] , to characterize m5C variance between two divergent schistosome lifecycle stages. Principal coordinate analysis (PCA, Fig. 1d , dotted versus solid circles) revealed clear separation of MSAP profiles between cercariae (water-dwelling) and adult worms (mammalian host residing) when parasite gDNA was restricted with methylation-sensitive Hpa II (an enzyme that cannot restrict C 5m /CGG) but not with the methylation insensitive isoschizomer Msp I (an enzyme that can restrict C 5m /CGG). These data suggested that some of the detected genomic m5C ( Fig. 1a,b ) was found in the context of CpG dinucleotide motifs and critically provides evidence that schistosomes alter their epigenome in response to different environmental stimuli. Finally, we extended our global analysis of schistosome DNA methylation to the identification of specific genomic loci that are modified by this epigenetic process. Among several cercarial gDNA fragments that were isolated by methyl cytosine enrichment, we chose to verify the presence of m5C in one particular locus by bisulfite conversion, bisulfite PCR and sequencing ( Fig. 2 ). This 316-bp locus (NCBI accession number JF781495) mapped to a highly repetitive intragenic intron within a predicted forkhead protein, Smp_155010 ( Fig. 2a ). Particular features of this methylated locus included a higher-than-genome-, scaffold (scaff000180)- or gene (Smp_155010)-%GC average ( Fig. 2b ) and detectable m5C in the context of CpG and CpA ( Fig. 2c ). Although detection of CpG methylation confirmed the MSAP studies ( Fig. 1d ), CpA methylation represents an additional feature of the schistosome epigenome. CpA dinucleotide motifs are also found methylated in other invertebrate species (for example, D. melanogaster [23] ) and suggest that the diversity of DNA methylation targets within the schistosome genome is not restricted to the CpG context. Importantly, the hypermethylation of a repetitive DNA element may indicate that the schistosome DNA methylation machinery has evolved to help silence or destroy these highly prevalent (and sometimes transcribed [24] ) parasitic genomic features as previously demonstrated in D. melanogaster [25] and Dictyostelium discoideum [26] , [27] . Complete sequencing of the schistosome epigenome will shed light on this hypothesis. 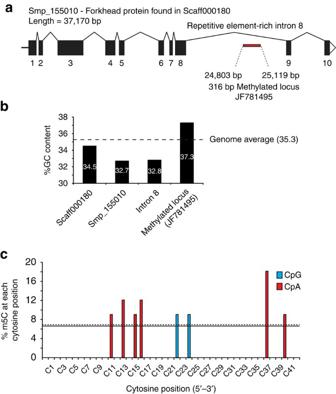Figure 2:S.mansoniforkhead protein contains a highly methylated intragenic intron. (a) Smp_155010 (ten exons—solid blocks, sequentially numbered and nine introns—black lines) is a predicted 37,170 bp gene encoding a forkhead protein found in scaff000180 of genome assembly 4.0. A m5C enrichment protocol initiated with cercarial gDNA yielded a highly methylated 316 bp locus, NCBI accession number JF781495 (red box; mapping to a repetitive element-rich region spanning 24,803–25,119 bp of intron 8), found within Smp_155010. (b) %GC representation ofS.mansonigenomic elements containing the methylated locus. (c) Enumeration of m5C abundance (dinucleotide context percentages) in clones (n=33) derived from bisulfite-PCR amplification of JF781495 after bisulfite cercarial gDNA conversion. The 42 cytosine positions within the 199-bp PCR product are indicated on the abscissa (5′–3′). Solid line represents mean false m5C discovery rate (FDR) derived from control bisulfite reactions (Methods) and dotted line represents mean FDR+3×s.e.m. Figure 2: S.mansoni forkhead protein contains a highly methylated intragenic intron. ( a ) Smp_155010 (ten exons—solid blocks, sequentially numbered and nine introns—black lines) is a predicted 37,170 bp gene encoding a forkhead protein found in scaff000180 of genome assembly 4.0. A m5C enrichment protocol initiated with cercarial gDNA yielded a highly methylated 316 bp locus, NCBI accession number JF781495 (red box; mapping to a repetitive element-rich region spanning 24,803–25,119 bp of intron 8), found within Smp_155010. ( b ) %GC representation of S.mansoni genomic elements containing the methylated locus. ( c ) Enumeration of m5C abundance (dinucleotide context percentages) in clones ( n =33) derived from bisulfite-PCR amplification of JF781495 after bisulfite cercarial gDNA conversion. The 42 cytosine positions within the 199-bp PCR product are indicated on the abscissa (5′–3′). Solid line represents mean false m5C discovery rate (FDR) derived from control bisulfite reactions (Methods) and dotted line represents mean FDR+3×s.e.m. Full size image DNA methylation components are coregulated in development Having provided mutually supportive confirmation for the presence of m5C (in the context of CpG and CpA dinucleotide motifs), we next interrogated the current S. mansoni genome assembly [28] for putative DNA methylation machinery components. Using the M. musculus DNA methyltransferase (Dnmt) 2 amino-acid sequence (AF0458899) as a query, we identified a single candidate S. mansoni DNA methyltransferase (Smp_145390; the only genome hit with E value <1e −5 ) following BLASTp analysis of the annotated schistosome genome ( Supplementary Table S1 ). Confirmation of this genome prediction by PCR-based complementary DNA cloning (derived from adult female worm RNA) revealed the presence of two alternatively spliced products (GenBank, accession numbers HM991456 and HM991457 , differing by a 24 base indel). Although both schistosome transcripts encoded proteins containing conserved carboxy-terminal methyltransferase catalytic domains, they both lacked the extended amino-terminal regulatory regions found among metazoan Dnmt1 and Dnmt3 family members [29] . With this observation in mind, we infer that the identified schistosome Dnmt orthologs are likely to be novel Dnmt2 family members [30] ( Supplementary Table S2 ). Therefore, we have named the protein products SmDnmt2 isoforms 1 and 2. Dnmt2 proteins, highly conserved across protists, plants, fungi and animals [30] , are enigmatic DNA methyltransferases as they can additionally harbour RNA methyltransferase activities [31] . Thus, in organisms that also contain the maintenance Dnmt1 and de novo Dnmt3 family members (for example, H. sapiens ), Dnmt2 is not the primary DNA methyltransferase responsible for genome methylation [32] . However, in organisms that only contain a Dnmt2 ortholog, clear evidence from D. melanogaster [23] , D. discoideum [27] and Entamoeba histolytica [33] indicates that these enzymes are relevant DNA methyltransferases. Pristionchus pacificus [34] and Schizosaccharomyces pombe [35] are notable exceptions to this rule as both organisms contain Dnmt2 orthologs, but lack a methylated genome. Deleterious mutations in the Dnmt2 methyltransferase catalytic domains are sufficient to prevent genome methylation in these species. Therefore, the presence of a single DNA methyltransferase, containing a fully conserved methyltransferase catalytic domain, in the schistosome genome implies that this enzyme (SmDnmt2) may be responsible for the DNA methylation detected ( Figs 1 and 2 ). This hypothesis was tested by post-transcriptional gene silencing (PTGS) of SmDnmt2 in adult worms ( Fig. 3 ). Small interfering RNA (siRNA)-mediated PTGS of SmDnmt2 led to a 75% reduction in the amount of detectable transcript compared with control worms treated with siRNAs for luciferase ( Fig. 3a ). The effect that SmDnmt2 knockdown had on global DNA methylation was subsequently assessed by MSAP analysis of adult worm gDNA and AMOVA (analysis of molecular variance) [36] . Worms treated with SmDnmt2 siRNA demonstrated a statistically significant (AMOVA analysis, P =0.008) decreased epigenetic distance (Φ PT , solid histograms) among Hpa II-digested populations (compared with luciferase siRNA control-treated worms) indicating a loss of DNA methyltransferase activity ( Fig. 3b ). The loss of differential MSAP products (between isoschizomers) following SmDnmt2 silencing was clearly indicative of a widespread decline in genome-wide methylation (for example, arrow in Fig. 3c , retention of 209 bp Hpa II gDNA peak in siSmDnmt2-silenced worms). Loss of m5C methylation within JF781495 (the methylated locus found in cercariae gDNA, Fig. 2 ) following SmDnmt2 silencing provides further evidence that the decline in global genome methylation is additionally observed within a specific locus targeted by the DNA methylation machinery ( Fig. 3d ). Low-level SmDnmt2 expression (25%) provides the most plausible explanation for the detection of residual methylation (that is, differential MSAP loci between isoschizomers or unaffected cytosine positions within JF781495) in siSmDnmt2-treated worms. Nevertheless, we contend that these PTGS experiments fully support the role of this gene product as a functional DNA methyltransferase. Additional SmDnmt2 activities, if any, are currently being sought. 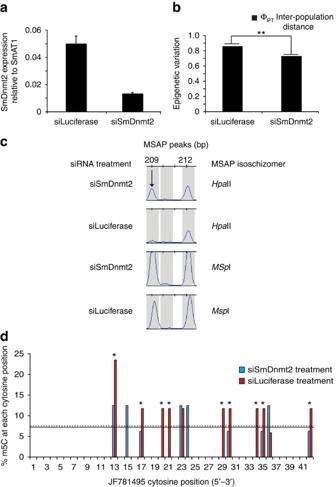Figure 3: SmDnmt2 is a functional DNA methyltransferase. Adult schistosome pairs (five pairs per treatment) were electroporated with siRNAs directed against SmDnmt2 or luciferase (negative control) according to the Methods section. (a) Quantitative real-time reverse transcription PCR (qRT–PCR) was used to assess the efficiency of SmDnmt2 silencing at 48 h post electroporation. All reactions were performed in triplicate (from biologically replicated samples,n=2) and SmDnmt2 expression was normalized to α-tubulin, SmAT1. Error bars represent the standard error of the normalized means (s.e.m.). Results are representative of three independent experiments. (b) AMOVA analysis of MSAP profiles was used to assess the degree of CpG cytosine methylation loss after 96 h post electroporation (five biologically replicated male samples/siRNA treatment). Epigenetic variation betweenHpaII peaks derived from siSmDnmt2-treated worms compared withHpaII peaks derived from siLuciferase-treated worms is statistically significant (AMOVA analysis, **P=0.008). (c) GeneMapper representation of an adult schistosome locus (arrow) where cytosine methylation is lost (loss ofHpaII sensitivity) upon SmDnmt2 silencing.MspI/HpaII represent the isoschizomers used to restrict gDNA before MSAP analysis. (d) Enumeration of m5C abundance (percentages) in 33 clones (siSmDnmt2,n=16; siLuciferase,n=17) derived from bisulfite-PCR amplification of JF781495 after bisulfite conversion of adult worm gDNA. The 42 cytosine positions within the 199 bp PCR product are indicated on the abscissa (5′–3′). Solid line represents mean false m5C discovery rate (FDR) derived from control bisulfite reactions and dotted line represents FDR mean+3×s.e.m. *Indicates the cytosine positions affected by SmDnmt2 silencing. Figure 3: SmDnmt2 is a functional DNA methyltransferase. Adult schistosome pairs (five pairs per treatment) were electroporated with siRNAs directed against SmDnmt2 or luciferase (negative control) according to the Methods section. ( a ) Quantitative real-time reverse transcription PCR (qRT–PCR) was used to assess the efficiency of SmDnmt2 silencing at 48 h post electroporation. All reactions were performed in triplicate (from biologically replicated samples, n =2) and SmDnmt2 expression was normalized to α-tubulin, SmAT1. Error bars represent the standard error of the normalized means (s.e.m.). Results are representative of three independent experiments. ( b ) AMOVA analysis of MSAP profiles was used to assess the degree of CpG cytosine methylation loss after 96 h post electroporation (five biologically replicated male samples/siRNA treatment). Epigenetic variation between Hpa II peaks derived from siSmDnmt2-treated worms compared with Hpa II peaks derived from siLuciferase-treated worms is statistically significant (AMOVA analysis, ** P =0.008). ( c ) GeneMapper representation of an adult schistosome locus (arrow) where cytosine methylation is lost (loss of Hpa II sensitivity) upon SmDnmt2 silencing. Msp I/ Hpa II represent the isoschizomers used to restrict gDNA before MSAP analysis. ( d ) Enumeration of m5C abundance (percentages) in 33 clones (siSmDnmt2, n =16; siLuciferase, n =17) derived from bisulfite-PCR amplification of JF781495 after bisulfite conversion of adult worm gDNA. The 42 cytosine positions within the 199 bp PCR product are indicated on the abscissa (5′–3′). Solid line represents mean false m5C discovery rate (FDR) derived from control bisulfite reactions and dotted line represents FDR mean+3×s.e.m. *Indicates the cytosine positions affected by SmDnmt2 silencing. Full size image A similar search was conducted for potential schistosome products that exhibited sequence similarity to methyl-CpG-binding domain (MBD) containing proteins. Instrumental to the DNA methylation machinery, these proteins are recruited to methylated DNA sequences and are thought to associate with a range of interacting partners to mediate transcriptional regulation [37] . BLASTp analysis of the schistosome genome with M. musculus MBD1 (NP_038622) as the query sequence identified one candidate schistosome MBD, Smp_138180 ( Supplementary Table S1 ; the only genome hit with E value <1e −05 ). Subsequent PCR-based cDNA cloning of this candidate schistosome MBD ortholog (derived from adult female mRNA) revealed a single product (SmMBD, HM991455), encoding a protein with an N-terminal methyl-binding domain and likely to be related to the conserved MBD2/3 ancestral protein [38] ( Supplementary Table S3 ). We hypothesized that if both SmDnmt2 and SmMBD were components of a functional DNA methylation machinery they would be transcriptionally coregulated during schistosome development. Quantitative real-time reverse transcription PCR (qRT–PCR) analysis of SmDnmt2 and SmMBD from schistosome lifecycle stages supported this hypothesis and indeed indicated coregulation of both transcripts during parasite development ( Fig. 4a ). Transcriptional regulation of SmDnmt2 mirrored the differential detection of m5C across the schistosome lifecycle ( Fig. 1b ) suggesting a direct link between the functional parasite gene product and this epigenetic modification. Furthermore, it was clear that both SmDnmt2 and SmMBD were more highly expressed in intra-molluscan developmental forms when compared with intra-mammalian forms and that these genes were already abundantly transcribed in the infective cercariae and miracidia lifecycle stages. It was also evident that sexually mature adult females expressed greater quantities of each transcript when compared with sexually mature adult males. Importantly, measurement of nuclear DNA methyltransferase activity in adult females and males confirmed the SmDnmt2 transcriptional results obtained from this lifecycle stage ( Fig. 4b ), supported the differential detection of m5C between gender ( Fig. 1b ) and verified the nuclear localization of a DNA methyltransferase activity responsible for m5C modifications in schistosomal cytological spreads ( Fig. 1c ). 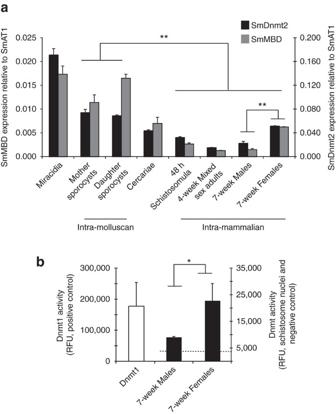Figure 4: SmDnmt2 and SmMBD are transcriptionally coregulated during schistosome development. (a) qRT–PCR determination of SmDnmt2- (black histograms) and SmMBD- (grey histograms) expression across the schistosome lifecycle. All reactions were performed in triplicate and SmDnmt2 and SmMDB expression were independently normalized to α-tubulin, SmAT1 (left ordinate=SmMBD/SmAT1; right ordinate=SmDnmt2/SmAT1). Error bars represent standard error of the normalized means (s.e.m.). A one-way analysis of variance (ANOVA) followed bypost hoctesting with Fisher's Least Significant Difference (LSD) was used to detect statistical differences (**P<0.001) in normalized gene expression between lifecycle stages. Intra-molluscan—schistosome life stages developing within the intermediate host; Intra-mammalian—parasite life stages developing within the definitive host. (b) DNA methyltransferase activity measured in adult female and male schistosome nuclei (relative fluorescence units (RFU) at excitation=530 nm and emission=590 nm). Dashed line represents background DNA methyltransferase activity (negative control). Left ordinate scale represents DNA methyltransferase activity obtained from the positive Dnmt1 control (n=2 biological replicates) and right ordinate scale represents DNA methyltransferase activity of parasite or negative control samples (n=2 biological replicates). Error bars represent the s.d. A one-way ANOVA followed bypost hoctesting with Fisher's LSD was used to detect statistical differences (*P<0.05) between gender. Figure 4: SmDnmt2 and SmMBD are transcriptionally coregulated during schistosome development. ( a ) qRT–PCR determination of SmDnmt2- (black histograms) and SmMBD- (grey histograms) expression across the schistosome lifecycle. All reactions were performed in triplicate and SmDnmt2 and SmMDB expression were independently normalized to α-tubulin, SmAT1 (left ordinate=SmMBD/SmAT1; right ordinate=SmDnmt2/SmAT1). Error bars represent standard error of the normalized means (s.e.m.). A one-way analysis of variance (ANOVA) followed by post hoc testing with Fisher's Least Significant Difference (LSD) was used to detect statistical differences (** P <0.001) in normalized gene expression between lifecycle stages. Intra-molluscan—schistosome life stages developing within the intermediate host; Intra-mammalian—parasite life stages developing within the definitive host. ( b ) DNA methyltransferase activity measured in adult female and male schistosome nuclei (relative fluorescence units (RFU) at excitation=530 nm and emission=590 nm). Dashed line represents background DNA methyltransferase activity (negative control). Left ordinate scale represents DNA methyltransferase activity obtained from the positive Dnmt1 control ( n =2 biological replicates) and right ordinate scale represents DNA methyltransferase activity of parasite or negative control samples ( n =2 biological replicates). Error bars represent the s.d. A one-way ANOVA followed by post hoc testing with Fisher's LSD was used to detect statistical differences (* P <0.05) between gender. Full size image Cytosine methylation regulates oviposition We next wanted to determine whether there is a functional role for cytosine methylation during platyhelminth development. As eggs are primarily responsible for most pathological changes in infected individuals and are responsible for lifecycle transmission in endemic areas, we elected to examine the role of cytosine methylation in the important process of schistosome oviposition. Moreover, linking cytosine methylation to egg production could provide valuable insights into this critical developmental process and crucially, identify useful targets for disease intervention strategies. The experimental approach chosen involved culturing adult worm pairs for 48 h in the continuous presence of the DNA methyltransferase inhibitors, 5-azacytidine (5-AzaC, a ribonucleoside) and 2′-deoxy-5-azacytidine (DAC or decitabine, a deoxyribonucleoside; Fig. 5 ) [39] . Both nucleoside analogues are integrated into replicating DNA where they form covalent bonds with Dnmts. This trapping of Dnmts triggers DNA damage signalling, Dnmt degradation and loss of methylation during subsequent rounds of DNA replication and cell division [40] . Whereas DAC preferentially incorporates into DNA, 5-AzaC also becomes incorporated into newly synthesized RNAs [41] and can affect the synthesis/turnover of proteins [42] . Because of these nucleoside-specific characteristics and due to the fact that neither 5-AzaC nor DAC have ever been tested on multi-cellular parasitic worms, it was first necessary to determine which compound was most effective in demethylating the adult schistosome genome. As both 5-AzaC and DAC are the FDA approved chemotherapies [43] used to induce selective toxicity in preleukemic bone marrow cells [44] , we first determined whether these nucleosides could directly kill adult schistosomes. Using bright-field microscopy and our recently developed helminth fluorescence bioassay [45] , we demonstrated that neither 5-AzaC nor DAC was lethal to adult worms (compared with controls), even when drug concentrations reached the limits of aqueous solubility (491 μM; Fig. 5a ). Although toxicity may develop with time, this observation allowed us to examine the effect of both 5-AzaC and DAC on cytosine methylation in viable adult schistosomes cultured for 48 h. Adult males, as opposed to adult females, were specifically chosen for this analysis because they do not contain m5C-rich egg gDNA ( Fig. 1b , compare m5C levels in male, female and egg gDNA), which greatly simplified our interpretation of each nucleoside's potential for reducing genomic cytosine methylation at the organism level. Using MSAP analysis of adult male gDNA and quantified by AMOVA, we show that 5-AzaC was more effective than DAC in decreasing epigenetic distance (Φ PT , solid histograms) among Msp I- and Hpa II-digested populations ( Fig. 5b ). Moreover, increased epigenetic variation was preferentially detected within 5-AzaC-treated populations (Φ RT , open histograms) reflecting the random nature of methylation loss selectively induced by 5-AzaC (when compared with DAC) on the genomes in each cell of a multi-cellular adult schistosome. Examples of MSAP Hpa II loci affected by 5-AzaC, but not by DAC, are illustrated to support the AMOVA analysis (dashed arrows in Fig. 5c ). On the basis of these results, 5-AzaC was chosen as the nucleoside analogue for further analyses on parasite genome methylation and oviposition. 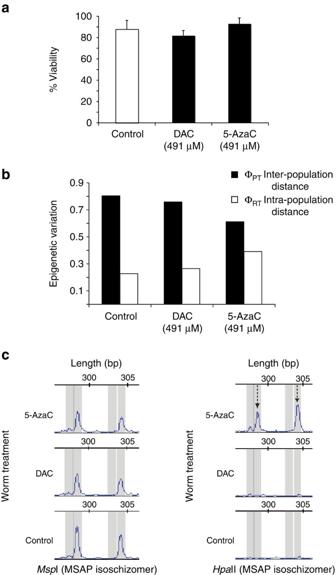Figure 5: Schistosome cytosine methylation is affected by 5-azacytidine (5-AzaC) but not decitabine (DAC). (a) The helminth fluorescent bioassay indicated that neither 5-AzaC nor DAC was toxic to adult male schistosomes (open histogram—% mean viability of control adult worms; filled histogram—% mean viability of adult worms treated with either 491 μM 5-AzaC or 491μM DAC). Error bars represent standard error of the normalized % viability mean (s.e.m.) collected from three individual worms. (b) AMOVA analysis of MSAP profiles was used to assess the degree of cytosine methylation loss after 48 h treatment with 5-AzaC (n=4 adult male biological replicates) and DAC (n=4 adult male biological replicates) compared with controls (n=4 adult male biological replicates). (c) GeneMapper representation of two adult male schistosome loci (dashed arrows) where CpG cytosine methylation is lost (loss inHpaII sensitivity) upon 5-AzaC, but not DAC, treatment.MspI/HpaII represent the isoschizomers used to restrict gDNA before MSAP analysis. Figure 5: Schistosome cytosine methylation is affected by 5-azacytidine (5-AzaC) but not decitabine (DAC). ( a ) The helminth fluorescent bioassay indicated that neither 5-AzaC nor DAC was toxic to adult male schistosomes (open histogram—% mean viability of control adult worms; filled histogram—% mean viability of adult worms treated with either 491 μM 5-AzaC or 491μM DAC). Error bars represent standard error of the normalized % viability mean (s.e.m.) collected from three individual worms. ( b ) AMOVA analysis of MSAP profiles was used to assess the degree of cytosine methylation loss after 48 h treatment with 5-AzaC ( n =4 adult male biological replicates) and DAC ( n =4 adult male biological replicates) compared with controls ( n =4 adult male biological replicates). ( c ) GeneMapper representation of two adult male schistosome loci (dashed arrows) where CpG cytosine methylation is lost (loss in Hpa II sensitivity) upon 5-AzaC, but not DAC, treatment. Msp I/ Hpa II represent the isoschizomers used to restrict gDNA before MSAP analysis. Full size image Further investigations into the ability of 5-AzaC ability to reduce methylation of the schistosome genome revealed a clear dose-dependent effect ( Fig. 6 ). Using MSAP analysis of adult male gDNA (free from host gDNA contamination, Fig. 6a ) and quantified by PCA ( Fig. 6b ) and AMOVA ( Fig. 6c ), increasing concentrations of 5-AzaC (0, 10 and 491 μM) led to a decrease in epigenetic distance (Φ PT , solid histograms) among Msp I- and Hpa II-digested populations. In addition, increased epigenetic variation was also detected within treated populations (Φ RT , open histograms) reflecting the dose-dependent random nature of methylation loss induced by 5-AzaC. 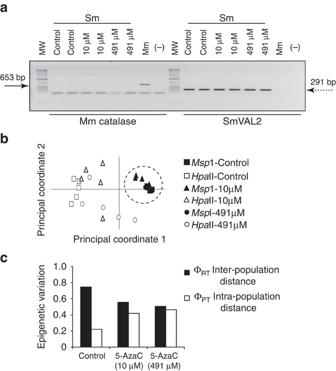Figure 6: 5-Azacytidine inhibitsS. mansoniDNA methylation in a dose-dependent manner. (a) Adult schistosome gDNA isolated from adult male worm cultures (control, 10 μM 5-AzaC and 491 μM 5-AzaC) were examined for the presence ofM. musculusgDNA contamination by PCR before MSAP analyses. Primers designed to amplifyM. musculus(Mm) catalase andS. mansoni(Sm) Venom Allergen Like (VAL) 2 were used. Mm catalase primers only amplified a product (sequence verified catalase, 653 bp, solid arrow) when Mm gDNA was used as a template. SmVAL2 primers only amplified a product (sequence verified SmVAL2, 291 bp, dashed arrow) when Sm gDNA was used as a template. (−) represents PCR conditions when no gDNA was included in the reaction and MW represents molecular weight standards. (b) MSAP analysis of m5C in gDNA obtained from 5-AzaC-treated adult male worms.HpaII (open shapes) andMspI (filled shapes enclosed by dashed circle) isoschizomers were used to restrict adult worm gDNA from control samples (squares), 10-μM 5-AzaC-treated samples (triangles) and 491-μM 5-AzaC-treated samples (circles). Five biological replicates were analysed for all treatments/enzyme combinations. The dose-dependent demethylating ability of 5-AzaC is illustrated by principal coordinate analysis. (c) Statistical assessment of MSAP profiles by AMOVA. Significant differences (P<0.01) in epigenetic variation are found between populations (ΦPT;HpaII-MspI inter-population distances between controls, 10 μM- and 491 μM-5-AzaC samples) and within populations (ΦRT;HpaII intra-population distances among controls compared withHpaII intra-population distances among 5-AzaC-treated worms). Figure 6: 5-Azacytidine inhibits S. mansoni DNA methylation in a dose-dependent manner. ( a ) Adult schistosome gDNA isolated from adult male worm cultures (control, 10 μM 5-AzaC and 491 μM 5-AzaC) were examined for the presence of M. musculus gDNA contamination by PCR before MSAP analyses. Primers designed to amplify M. musculus (Mm) catalase and S. mansoni (Sm) Venom Allergen Like (VAL) 2 were used. Mm catalase primers only amplified a product (sequence verified catalase, 653 bp, solid arrow) when Mm gDNA was used as a template. SmVAL2 primers only amplified a product (sequence verified SmVAL2, 291 bp, dashed arrow) when Sm gDNA was used as a template. (−) represents PCR conditions when no gDNA was included in the reaction and MW represents molecular weight standards. ( b ) MSAP analysis of m5C in gDNA obtained from 5-AzaC-treated adult male worms. Hpa II (open shapes) and Msp I (filled shapes enclosed by dashed circle) isoschizomers were used to restrict adult worm gDNA from control samples (squares), 10-μM 5-AzaC-treated samples (triangles) and 491-μM 5-AzaC-treated samples (circles). Five biological replicates were analysed for all treatments/enzyme combinations. The dose-dependent demethylating ability of 5-AzaC is illustrated by principal coordinate analysis. ( c ) Statistical assessment of MSAP profiles by AMOVA. Significant differences ( P <0.01) in epigenetic variation are found between populations (Φ PT ; Hpa II- Msp I inter-population distances between controls, 10 μM- and 491 μM-5-AzaC samples) and within populations (Φ RT ; Hpa II intra-population distances among controls compared with Hpa II intra-population distances among 5-AzaC-treated worms). Full size image Having demonstrated that 5-AzaC inhibits cytosine methylation in adult schistosomes ( Figs 5 and 6 ), we next investigated whether deficiencies in this epigenetic process affected egg production, egg phenotype, egg maturation and ovarian morphology ( Fig. 7 ). Treatment of adult worm pairs with 5-AzaC led to a reduction in female egg output over a 48-h period when compared with control worms ( Fig. 7a ) or worm pairs treated with DAC ( Supplementary Fig. S1 ). This observation was dose dependent, correlated to the degree of genome demethylation ( Figs 5 and 6 ) and statistically significant even when 5-AzaC concentrations were as low as 10 μM. Although eggs laid by control female worms were phenotypically normal (oval, presence of a lateral spine, regular auto-fluorescence due to eggshell tanning [46] and ∼ 150 μm in length), eggs laid by 5-AzaC-treated females displayed a broad range of phenotypic abnormalities ( Fig. 7b ). These abnormal eggs included individuals that lacked lateral spines, were often much smaller than controls (as small as 50 μm), were spherical rather than oval and were not fully hardened or tanned (irregularly autofluorescent). Eggs displaying more than one of these phenotypes were the norm and were additionally observed within the uterus ( Fig. 7c ), which indicated that 5-AzaC's inhibition of cytosine methylation had disrupted several vital components of the schistosome oviposition pathway. 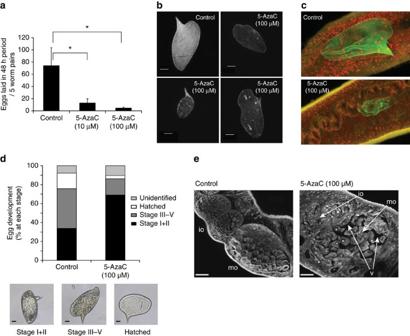Figure 7: Schistosome egg development and ovarian architecture are regulated by cytosine methylation. (a) 5-Azacytidine (5-AzaC) inhibits egg production in a dose-dependent manner. Histograms represent mean (+s.e.m.) egg output derived from five worm pairs (n=4) cultured for 48 h. A one-way analysis of variance (ANOVA) followed bypost hoctesting with Fisher's Least Significant Difference (LSD) was used to detect statistical differences (*P<0.05) in egg production among groups (control, 10 μM 5-AzaC and 100 μM 5-AzaC). Data are derived from a representative experiment (replicated five times). (b) Confocal microscopy of schistosome eggs laid by control worm pairs (control) or 5-AzaC-treated worm pairs (5-AzaC, 100 μM). Scale bar, 20 μm. (c) Confocal microscopy of normal adult females (control) or 5-AzaC-treated females (5-AzaC, 100 μM) stained with Langeron's Carmine and imaging focused on a region containing the intra-uterine egg. Scale bar, 20 μm. (d) 5-AzaC inhibits egg development as assessed byin vitrostaging. Eggs deposited by control females (control) or 5-AzaC-treated females (5-AzaC, 100 μM) were left to develop as described in the Methods section and maturation classified according to four categories (stage I+II, stage III−V, hatched or unidentified; scale bar, 20 μm). The percentage of eggs displaying each developmental stage is indicated by a stacked histogram and is representative of two independent experiments. (e) Confocal microscopy of normal adult females (control) or 5-AzaC-treated females (5-AzaC, 100 μM) stained with Langeron's Carmine and imaging focused on a region containing the ovary. Scale bar, 20 μm. Io, immature oocyte; mo, mature oocyte; v, vacuole. Figure 7: Schistosome egg development and ovarian architecture are regulated by cytosine methylation. ( a ) 5-Azacytidine (5-AzaC) inhibits egg production in a dose-dependent manner. Histograms represent mean (+s.e.m.) egg output derived from five worm pairs ( n =4) cultured for 48 h. A one-way analysis of variance (ANOVA) followed by post hoc testing with Fisher's Least Significant Difference (LSD) was used to detect statistical differences (* P <0.05) in egg production among groups (control, 10 μM 5-AzaC and 100 μM 5-AzaC). Data are derived from a representative experiment (replicated five times). ( b ) Confocal microscopy of schistosome eggs laid by control worm pairs (control) or 5-AzaC-treated worm pairs (5-AzaC, 100 μM). Scale bar, 20 μm. ( c ) Confocal microscopy of normal adult females (control) or 5-AzaC-treated females (5-AzaC, 100 μM) stained with Langeron's Carmine and imaging focused on a region containing the intra-uterine egg. Scale bar, 20 μm. ( d ) 5-AzaC inhibits egg development as assessed by in vitro staging. Eggs deposited by control females (control) or 5-AzaC-treated females (5-AzaC, 100 μM) were left to develop as described in the Methods section and maturation classified according to four categories (stage I+II, stage III−V, hatched or unidentified; scale bar, 20 μm). The percentage of eggs displaying each developmental stage is indicated by a stacked histogram and is representative of two independent experiments. ( e ) Confocal microscopy of normal adult females (control) or 5-AzaC-treated females (5-AzaC, 100 μM) stained with Langeron's Carmine and imaging focused on a region containing the ovary. Scale bar, 20 μm. Io, immature oocyte; mo, mature oocyte; v, vacuole. Full size image After establishing that there is an important role for cytosine methylation in normal egg output/phenotype, we investigated whether this epigenetic process regulated the in vitro developmental maturation of newly deposited eggs ( Fig. 7d ). According to the staging classification of Michaels and Prata [47] , schistosome eggs undergo a process of in vitro development involving five discrete forms (stages I–V; representative stage I+II, stage III–V and hatched eggs are illustrated in Fig. 7d ). Although development of eggs proceeded normally in control wells over a 6-day period, egg maturation was markedly impaired in wells containing 5-AzaC. Very few eggs released miracidia (3% hatched eggs compared with 16% found in control wells) and most ( ∼ 70% compared with 33% found in control wells) never progressed past stage I+II (embryonic disk occupying one half of the diameter of the egg). Together, these results firmly indicated that cytosine methylation also influences normal egg developmental progression and, thus, probably has a significant role in schistosomiasis transmission. Finally, our attention was drawn to the effect that 5-AzaC had on ovarian morphology within cultured female schistosomes ( Fig. 7e ). S. mansoni females each contain one ovary, where small, poorly differentiated immature oocytes develop into well-differentiated mature oocytes along an anterior to posterior gradient. Whereas this organization was consistently observed in control female worms, 5-AzaC-treated females contained reproducible gross-morphological defects including numerous large inter-mo vacuoles, atypical dendritic-like process extending into the vacuoles and a complete breakdown in normal ovarian architecture. Although we have yet to determine how these abnormalities influence zygote formation and egg production, we contend that cytosine methylation and SmDnmt2 are instrumental in the uniform gradient of oocyte development within the ovary and mo release into the oviduct. Together with a role in eggshell tanning, egg production and maturation, our results strongly suggest that cytosine methylation participates in most major aspects of schistosome oviposition. Less than 3 years after the S. mansoni genome was reported [28] and 10 years after the failure to detect DNA methylation [8] , a functional role for m5C modifications during oviposition has been established ( Fig. 7 ). This discovery represents a significant advance in our understanding of platyhelminth biology. Additional findings reported herein that illustrate a clear link between m5C abundance ( Fig. 1 ) and SmDnmt2 developmental expression ( Fig. 4 ) suggest an auxiliary role for the schistosome DNA methylation machinery in transitioning between free-living and parasitic life styles, worm maturation within the definitive mammalian host and sporocyst asexual processes (for example, multiplication of infective stage cercariae) within the intermediate snail host. Further mechanistic studies into how this particular epigenetic modification is influenced by diverse environmental stimuli (water, intermediate or definitive hosts) may ultimately shed new light on the fine nuances of host/parasite cross talk including orchestration of successful survival strategies, development of extended phenotypes and the induction of appropriate danger signals. The identification of all genomic loci differentially methylated during schistosome development (in addition to the single methylated locus found herein, Fig. 2 ) will help in this endeavour. Although we do not yet have an explanation for why 5-AzaC is more effective than DAC in reducing schistosome genome methylation ( Fig. 5 ), it is likely that the differential ability of these two nucleoside analogues to cross the parasite's outer heptalaminate membrane [48] or the differential stability of each during the in vitro cultivation period [40] , [49] may be responsible. Nevertheless, our data suggest that 5-AzaC is a stable inhibitor of DNA methyltransferase activity and is capable of inhibiting native SmDnmt2 (the only bona fide functional DNA methyltransferase in the schistosome genome, Supplementary Table S2 ; Fig. 3 ) during in vitro schistosome cultivation. Whether 5-AzaC or SmDnmt2 also affect schistosome RNA methylation [31] , [50] is currently unknown, but is the subject of ongoing investigations. We envisage that the discovery of this epigenetic alteration within an ancient invertebrate lineage will drive future investigations aimed at deciphering its contrasting and overlapping roles during metazoan evolution. Perhaps, more importantly in the context of schistosomiasis control, our results demonstrate that targeting parasite cytosine methylation components with selective demethylating agents present a promising new avenue through which to combat a major human neglected tropical disease. Parasite cultivation and gDNA isolation A Puerto Rican strain of S. mansoni was used in this study. All procedures performed on mice (6- to 7-week-old female Tuck Ordinary and C57BL/6 strains; Harlan, UK) adhered to the United Kingdom Home Office Animals (Scientific Procedures) Act of 1986 and were approved by Aberystwyth University's Ethical Review Panel. Parasite material was obtained as previously described [6] . When necessary, adult worms and schistosomula were cultured at 37 °C in DMEM supplemented with 10% foetal calf serum, 2 mM L -glutamine and 100 mg ml −1 penicillin/streptomycin in an atmosphere of 5% CO 2 for up to 48 h with a 70% media exchange performed after 24 h. Genomic DNA was isolated from parasite material using the Qiagen DNeasy Blood and Tissue Kit (Qiagen), with contaminating RNA eliminated using an RNase cocktail. GC–MS identification of m5C Derivatization of mixed-sex adult worm m5C and detection of m5C derivative by GC–MS was performed according to Crain [51] using a HP-1 MS GC column. Briefly, MS data were acquired using an Agilent 5973N GC/MS instrument (Agilent) operated in the selected ion-monitoring mode. The tert-butyldimethylsilyl m5C derivative was detected by measuring the intensity of the selected ion ( m / z =296.2) throughout the GC run. 5-AzaC and decitabine treatment of S. mansoni adults Adult worms were cultured at a density of ten worms (five male/female pairs or ten individuals of the same gender) per well in 1 ml of media and different concentrations of 5-AzaC or decitabine (DAC; Sigma-Aldrich). Each condition was performed in quadruplicate with the experiment replicated three to five times. After 48 h, the adult worms were removed, gender separated (if necessary), their viability determined and gDNA prepared for m5C detection. In wells containing adult worm pairs, the eggs were counted and subsequently subjected to laser confocal imaging. ELISA detection of m5C Cytosine methylation was fluorescently detected in S. mansoni gDNA samples (100 ng) using the DNA SuperSense Methylated DNA Quantification assay (Epigentek) following the manufacturer's instructions. Fluorescent values obtained from the negative DNA control sample (containing 0% m5C) were subtracted from the fluorescent readings obtained for all of the schistosome gDNA samples as well as the positive DNA control samples (containing 100% m5C). The adjusted fluorescence detected in the positive DNA control sample was now set to 100% (maximal detected m5C) and m5C abundance in each schistosome lifecycle stage was normalized to this value and depicted as a percentage. m5C immunolocalization and GISH of cytological preparations Cytological spreads were prepared from intra-molluscan parasites [52] . Slides, containing both Schistosoma and Biomphalaria nuclei, were incubated overnight at 4 °C with mouse anti-m5C primary Ab (Calbiochem, Clone 162 33 D3) or nonspecific anti-mouse IgG 1 (Invitrogen). GISH, to distinguish Schistosoma nuclei, was subsequently performed according to Hasterock et al . [53] Slides were finally incubated for 2 h at room temperature with Alexa Fluor 488 conjugated goat anti-mouse IgG secondary antibody (Invitrogen). Cytological spreads were counterstained with diamidio-2-phenylindole. MSAP analysis of S. mansoni CpG methylation To compare cytosine methylation patterns between schistosome samples, an AFLP (amplified fragment length polymorphism) protocol developed by Vos et al . [54] and modified for methylation analysis by Reyna-Lopez et al . [22] was employed. Each study used the isoschizomers Hpa II and Msp I as well as Eco RI. For lifecycle studies, seven mixed-sex adult- and cercarial-gDNA samples were used; for comparative drug studies, four adult male samples were used per condition (491 μM DAC, 491 μM 5-AzaC and controls); for 5-AzaC titration studies, five adult male samples were used for each condition (0, 10 and 491 μM 5-AzaC); for siRNA studies, five adult male samples were used for each treatment (siDnmt2- and siLuciferase-treated worms). Sample fractioning of fluorescently labelled MSAP products was performed on an ABI 3100 DNA Fragment Analyzer. Pairwise F ST (genetic variance among populations) and AMOVA [36] were subsequently calculated using GenAlex (v.6.4) to analyse the proportion of variance distributed among and within samples as well as to test the significance of F ST between samples [55] . The probability of non-differentiation ( F ST =0) was estimated over 9,999 permutations ( Fig. 3b ). Measurement of DNA methyltransferase activity DNA methyltransferase activity was measured in nuclear protein extracts processed from adult male and female worms cultured in vitro for 48 h. An EpiQuik™ Nuclear Extraction Kit I (Epigentek) was used to prepare the adult worm nuclear protein extracts while an EpiQuik DNA Methyltransferase Activity/Inhibition Kit (Epigentek) was used to quantify DNA methyltransferase activity. Methylated gDNA locus identification Methylated fragment enrichment (originating with cercariae gDNA) was performed using the Methylminer Methylated DNA Enrichment Kit (Invitrogen) according to the manufacturer's instructions. After sequencing 35 randomly chosen clones and mapping to the S. mansoni genome (assembly 4.0), one locus was selected (deposited under NCBI accession number JF781495, mapping to intron eight of Smp_105510; scaffold000180 position 213,627—213,942 bp) for methylation status confirmation by sodium bisulfite conversion using the BisulFlash DNA Modification Kit (Epigentek). Bisulfite PCR primers ( Supplementary Table S4 , designed using Methyl Primer Express v. 1.0, http://www.appliedbiosystems.com/ ) were used to amplify a 199 bp fragment of JF781495 from converted gDNA samples. Purified PCR products were cloned using the TOPO TA Cloning Kit (Invitrogen) and 33 clones subsequently sequenced, aligned and analysed for their methylation status. Cytosine methylation of this locus in adult samples was additional performed as part of the siRNA manipulations. Calculation of sodium bisulfite conversion efficiency Sodium bisulfite conversion efficiency was calculated using a non-methylated DNA control (741-bp PCR product derived from Smp_121930.1, NCBI accession number XM_002571391). This control sample was added to schistosome gDNA samples (derived from siRNA experiments) before sodium bisulfite conversion. Bisulfite-PCR amplification of the control sample after conversion generated a 386 bp amplicon (53 cytosines in the parent DNA molecule between bisulfite primer-binding sites; primer sequences found in Supplementary Table S4 ). Sequence analysis of the purified clones ( n =18) facilitated the quantification of sodium bisulfite conversion efficiency (93.5 and 93.3% in two independent reactions). Therefore, an average bisulfite conversion efficiency of 93.4% and a false positive m5C detection rate of 6.6% were detected in this study. Accordingly, we only report the C positions (and their dinucleotide context) within bisulfite-converted JF781495 that have a 6.9% non-conversion rate (mean false positive discovery rate+3×s.e.m.). These Cs represent the most likely methylated positions within the parent JF781495 sequence. RNA isolation and RT–PCR analysis S. mansoni total RNA isolation and qRT–PCR analyses was performed as previously described [6] , [56] . Briefly, all schistosome lifecycle stages used for qRT–PCR analysis were derived from cDNA reactions initiated by 1-μg total RNA (obtained from each profiled or siRNA manipulated lifecycle stage). Reverse transcriptase-negative control reactions were included in each experiment to account for gDNA contamination. All qRT–PCR amplifications were performed in triplicate using Fast SYBR Green chemistry and a StepOnePlus thermocycler (Applied Biosystems). qRT–PCR primers (sequences found in Supplementary Table S4 ), spanning introns where possible, were used for amplifying SmDnmt2 and SmMBD. SmDnmt2 and SmMBD gene expression results were independently normalized to α-tubulin (SmAT1, primer sequences found in Supplementary Table S4 ), a constitutively expressed house-keeping gene [6] . siRNA mediated SmDnmt2 silencing siRNAs, spanning the coding region of SmDnmt2 at positions 351–376 bp, were used to silence SmDnmt2. siRNAs designed for firefly luciferase functioned as a negative control. For each siRNA treatment, five adult worm pairs were electroporated as described elsewhere [57] . Each experimental condition was performed in duplicate and RNA was isolated from adult worm pairs after a 48 h in vitro culture period (see above). SmDnmt2 silencing was then assessed by qRT–PCR from technical triplicates as described above. To investigate whether SmDnmt2 silencing led to a loss in genome methylation, gDNA from siRNA-treated worm pairs (siSmDnmt2 and siLuciferase, five biological replicates for each) were isolated after a 96-h in vitro culture and MSAP analysis performed as described above. Viability assay The helminth fluorescent bioassay developed by Peak et al . [45] was used to assess the viability of adult schistosomes treated with 5-AzaC and DAC (at 491 μM). Three adult male schistosomes were used for each experimental manipulation. Assessment of egg development Adult worm pairs were removed from control and 5-AzaC-treated (100 μM) cultures after 48 h and the produced eggs were left to develop for a further 4 days. On day 6, eggs were transferred to artificial river water and exposed to a light source for 2 h to induce hatching. Afterwards, all material was fixed in 10% buffered formalin, enumerated and categorized into four groups according to their state of maturation [47] : stage I+II, stage III–V, hatched egg and unidentified. Carmine staining of adult female schistosomes Adult female worms were fixed in AFA (48% alcohol, 25% formalin, 2% acetic acid) and stained with Langeron's Carmine as previously described [58] . Parasite material was cleared with xylene and worms subsequently mounted with DPX (distyrene, plasticiser, xylene) before confocal microscopy. Confocal laser microscopy Carmine stained adult female worms and schistosome eggs deposited in vitro were examined with a Leica TCS SP5II confocal microscope. A ×40 immersion lens, a 488-nm argon laser and a 561-nm diode-pumped, solid state (DPSS) laser were used to examine the adult female worms. Eggs were fixed in 10% saline-buffered formalin and examined using a ×63 oil immersion lens and a 488-nm argon laser. Accession codes: Sequences corresponding to the S. mansoni DNA methylation machinery components and the 316 bp methylated DNA locus have been submitted to the GenBank Nucleotide database under the accession numbers HM991456 , HM991457 , HM991455 and JF781495 . How to cite this article: Geyer, K. K. et al . Cytosine methylation regulates oviposition in the pathogenic blood fluke Schistosoma mansoni . Nat. Commun. 2:424 doi: 10.1038/ncomms1433 (2011).